An improved monomeric infrared fluorescent protein for neuronal and tumour brain imaging Infrared fluorescent proteins (IFPs) are ideal for in vivo imaging, and monomeric versions of these proteins can be advantageous as protein tags or for sensor development. In contrast to GFP, which requires only molecular oxygen for chromophore maturation, phytochrome-derived IFPs incorporate biliverdin (BV) as the chromophore. However, BV varies in concentration in different cells and organisms. Here we engineered cells to express the haeme oxygenase responsible for BV biosynthesis and a brighter monomeric IFP mutant (IFP2.0). Together, these tools improve the imaging capabilities of IFP2.0 compared with monomeric IFP1.4 and dimeric iRFP. By targeting IFP2.0 to the plasma membrane, we demonstrate robust labelling of neuronal processes in Drosophila larvae. We also show that this strategy improves the sensitivity when imaging brain tumours in whole mice. Our work shows promise in the application of IFPs for protein labelling and in vivo imaging. The monomeric green and red fluorescent proteins (FPs) are powerful tools for multicolour protein labelling [1] , [2] , [3] . To add another labelling colour and to open the application to whole-animal fluorescence imaging, we previously engineered a bacterial phytochrome into a monomeric infrared fluorescent protein1.4 (IFP1.4) (refs 4 , 5 , 6 ). Because infrared light penetrates through tissue more efficiently than visible light [7] , [8] , IFP1.4 outperforms far-red FP in imaging studies of the liver in intact mice, even though the molecular brightness (quantum yield × extinction coefficient) of IFP1.4 is lower. Subsequently, another phytochrome-based IFP, near-infrared fluorescent protein (iRFP), was developed and was shown to have molecular brightness that is similar to IFP1.4 but to have significantly higher brightness in cells (cellular brightness) [9] . Moreover, although the molecular brightness of other far-red FPs with the green fluorescent protein (GFP) fold is higher, iRFP outperforms them in whole-animal imaging. iRFP is dimeric, however, that limits its application in protein labelling. We therefore decide to engineer a brighter monomeric IFP. Using directed evolution, we first improve the previously engineered monomeric IFP1.4 and name the new mutant IFP2.0, of which the cellular brightness is similar to iRFP. Because the chromophore of phytochrome-derived IFPs is converted from haeme by the haeme oxygenase 1 (HO1) and the activity of HO1 varies in different cells, we then engineer the cofactor biosynthetic pathway into cells and animals to further increase the brightness. Our work demonstrates that the engineered cofactor biosynthesis significantly improves cellular brightness of IFP2.0 in human glial cells, primary neurons from mice and peripheral neurons in intact Drosophila. The plasma membrane-targeted IFP2.0 (with HO1) successfully labels neuronal processes in Drosophila , whereas the plasma membrane-targeted iRFP fails with no detectable fluorescence in neuronal processes or soma. IFP2.0 and HO1 also improve tumour imaging in the intact mouse brain, compared with iRFP. Our method will thus be useful in in vivo imaging. Directed evolution of IFP2.0 During directed evolution of the bacterial phytochrome DrBphP to IFP1.4 ( Fig. 1a ), we observed that, while disruption of the dimer interface in dimeric IFP1.2 led to monomeric IFP1.3, it significantly decreased the cellular brightness. Further engineering of IFP1.3 to IFP1.4 rescued the cellular brightness. On the basis of this, we reasoned that, by combining the beneficial mutations of the dimeric IFP1.2 and the monomeric IFP1.4, we might be able to ‘breed’ a brighter monomeric mutant. Through DNA shuffling followed by random mutagenesis [10] , [11] , we developed the brighter, monomeric IFP2.0. IFP2.0 is slightly red-shifted with excitation and emission maxima at 690 and 711 nm, respectively ( Supplementary Fig. 1 ), compared with 684 and 708 nm for IFP1.4. 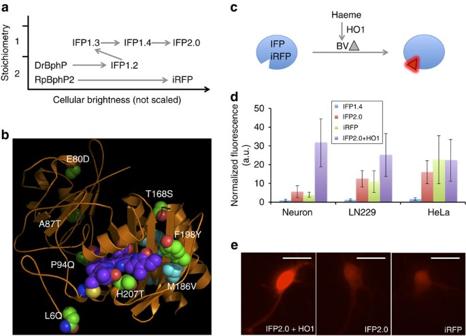Figure 1: Directed evolution of a bright and monomeric infrared fluorescent protein (IFP2.0) and engineering of its cofactor biosynthesis. (a) Schematic diagram showing directed evolution of IFP2.0. (b) Crystal structure of IFP2.0 at atomic resolution (1.14 Å). The mutations relative to IFP1.4 are labelled. Seven (in green) of 11 mutations are newly introduced, the remaining four (in cyan) are reverse mutations from IFP1.4 to IFP1.2. Three of these four are located at the c-terminus (barely seen behind the chromophore,Supplementary Fig. S3). BV is shown in purple. (c) Phytochrome-based IFPs and iRFP incorporate BV as the chromophore, which is an initial product of haeme by haeme oxygenase (HO1) and becomes fluorescent only when bound to IFPs. (d) Comparison of the cellular brightness of IFP1.4, IFP2.0, iRFP and IFP2.0+HO1 in three cell types: primary hippocampal neuron, glioma cell LN229 and cervical cancer cell HeLa. Fluorescence is normalized by coexpressed GFP. The error bar represents s.d. (n=10). (e) Representative fluorescence images of neurons showing significant increase in cellular brightness by coexpression of HO1. Scale bar, 40 μm. Although IFP2.0 has similar quantum yield and extinction coefficient as IFP1.4 ( Supplementary Table 1 ), it is significantly brighter (~13-fold, normalized to coexpressed GFP) when expressed in mammalian cells (HEK293) in the absence of exogenous biliverdin (BV) ( Supplementary Fig. 2a ). Sequence alignment of IFP2.0 with its ancestral forms: DrCBD (truncated form of DrBphP), IFP1.2 and 1.4, reveals several reverse mutations from IFP1.4 to 1.2, as well as several new mutations ( Supplementary Fig. 3 ). Since the cellular brightness is dependent on both molecular brightness and holoprotein concentration, our results suggest that the holo-IFP2.0 concentration is higher than holo-IFP1.4, perhaps due to increased protein solubility, stability and BV-binding affinity. iRFP has been shown to have similar characteristics [9] . Figure 1: Directed evolution of a bright and monomeric infrared fluorescent protein (IFP2.0) and engineering of its cofactor biosynthesis. ( a ) Schematic diagram showing directed evolution of IFP2.0. ( b ) Crystal structure of IFP2.0 at atomic resolution (1.14 Å). The mutations relative to IFP1.4 are labelled. Seven (in green) of 11 mutations are newly introduced, the remaining four (in cyan) are reverse mutations from IFP1.4 to IFP1.2. Three of these four are located at the c-terminus (barely seen behind the chromophore, Supplementary Fig. S3 ). BV is shown in purple. ( c ) Phytochrome-based IFPs and iRFP incorporate BV as the chromophore, which is an initial product of haeme by haeme oxygenase (HO1) and becomes fluorescent only when bound to IFPs. ( d ) Comparison of the cellular brightness of IFP1.4, IFP2.0, iRFP and IFP2.0+HO1 in three cell types: primary hippocampal neuron, glioma cell LN229 and cervical cancer cell HeLa. Fluorescence is normalized by coexpressed GFP. The error bar represents s.d. ( n =10). ( e ) Representative fluorescence images of neurons showing significant increase in cellular brightness by coexpression of HO1. Scale bar, 40 μm. Full size image Crystal structure of IFP2.0 While understanding the exact biophysical mechanisms will require further characterization, we solved the crystal structure of IFP2.0 at atomic resolution (1.14 Å), which so far is the highest resolution structure of proteins in the phytochrome family ( Fig. 1b , Supplementary Fig. 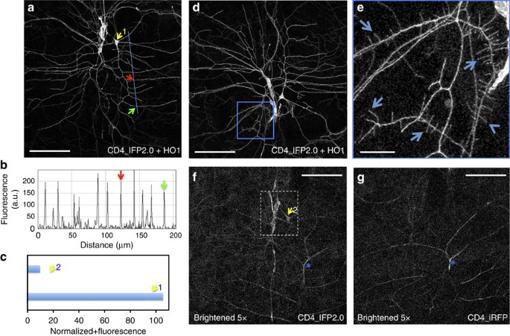Figure 2: IFP2.0 with engineered biosynthesis of the cofactor improves neuronal imaging inDrosophilalarvae Cellular membrane of dendritic arborization (da) neurons labelled by (a,d,e) IFP2.0 fused to CD4 with expression of HO1 that produces the cofactor (CD4-IFP2.0+HO1); (f) CD4-IFP2.0; (g) CD4-iRFP. (b) Fluorescence intensity profile along the line ina; the green and red arrows point to the dendrites ina. (c) Normalized fluorescence intensity of the cell body pointed by the yellow arrow inaandf. (e) Confocal image of the area (blue box) ind, with arrows pointing to dendritic spikes. Scale bar: (a,d,f,g), 100 μm; (e), 20 μm. 4 , Supplementary Table 2 ). The overall structure revealed that the protein scaffold was significantly evolved with root-mean-square deviation of atomic positions, 0.96 Å, between IFP2.0 and DrCBD (PDB entry code 2O9C) ( Supplementary Fig. 4b ). These changes resulted in a more compact structure of IFP2.0, which may have improved protein folding, solubility and stability. We located the eleven mutations in IFP2.0 relative to IFP1.4: one mutation (L6Q) is at the N-terminal loop; three mutations (E80D, A87T and P94Q) are in the PAS domain; and seven mutations (T168S, F198Y, H207T, M186V, E307Y, K311L and G314L) are in the GAF domain. Interestingly, four of the seven mutations in the GAF domain are reverse mutations from IFP1.4 to IFP1.2. Three mutations are near the chromophore (F198Y, H207T and M186V). H207 is the closest mutated residue to the chromophore, and the introduced His→Thr is a significant change. Therefore, H207T may be one of the key mutations responsible for the improved cellular brightness. Indeed, introduction of H207T into IFP1.4 improved the cellular brightness approximately threefold ( Supplementary Fig. 2b ), supporting the idea that this residue is an important one and suggesting that further improvement may be possible via saturation mutagenesis of this residue or other residues near this position. The crystal structure also provides potential mechanisms of engineered fluorescence of IFP1.4. Compared with the non-fluorescent DrCBD, one of the key mutations in IFP1.4 is A288V. V288 may function as a ‘clamp’ that locks up the third ring of the chromophore through van der Waals interaction ( Supplementary Fig. 4d–f ) and contributes to the fluorescence. Mutations at positions 195, 196 and 198 result in a cation-pi interaction between Arg172 and Tyr198, which rigidifies two β-strands in the vicinity of the fourth ring of the chromophore ( Supplementary Fig. 4b ) and most likely favours radiative decay of the chromophore’s excited state. Stoichiometry of IFP2.0 Size-exclusion chromatography indicates that IFP2.0 is monomeric ( Supplementary Fig. 5 ), although it retains only one (V318R) of the four mutations (Y307E, L311K, L314G and V318R) in IFP1.3 that are at the dimer interface of the wild-type protein DrCBD ( Supplementary Fig. 3 ). The crystal structure of IFP2.0 also revealed that the dimer interface present in DrCBD is no longer present in IFP2.0. These features suggest that V318R is sufficient to favour the monomeric form, a result that may be relevant to monomerizing other dimeric bacteriophytochrome-derived FPs such as iRFP. Engineering the cofactor biosynthesis pathway As noted above, the phytochrome-derived IFPs require the non-fluorescent BV as the cofactor ( Fig. 1c ). BV is the initial catabolic product of haeme by the haeme oxygenase (HO1). Its endogenous concentration is thus expected to vary over wide ranges between different cell types, depending on the activity of HO1. We analysed three different cell types in addition to the HEK293 line and found that the infrared fluorescence of all the IFPs (including IFP1.4, IFP2.0 and iRFP), which was normalized by coexpressed GFP, was the lowest in primary hippocampal neurons ( Fig. 1d ). The infrared fluorescence in HeLa cells was significantly higher than that in hippocampal neurons, and the fluorescence in the glial tumour cell line (glioblastoma) LN229 was intermediate ( Fig. 1d ). Because of its potential importance in neurobiology and the advantage that might be conferred by adding another colour to other FP-related methods such as the Brainbow technology that has been used to label different types of neurons [12] , we decided to engineer the cofactor biosynthetic pathway for robust infrared fluorescence in neurons. We first coexpressed HO1 with IFP2.0 in neurons and observed that the fluorescence of IFP2.0 increased to a level similar to that in HeLa ( Fig. 1d,e ). Coexpression of HO1 increased the cellular brightness of LN229 glial tumour cells by approximately twofold, but had no apparent effect on HeLa cells. These results suggest that engineering BV biosynthesis might overcome variations of endogenous BV concentration in different types of cells and can increase the utility and applicability of an IFP technology as a genetically encoded tag. We studied potential effects of HO1 expression in the primary neurons. First, we observed that cultured neurons that overexpress HO1 formed normal neuronal networks with no apparent differences compared with those without HO1 overexpression ( Supplementary Fig. 6 ). Second, we recorded electrophysiological properties of the neurons expressing IFPs and found no differences in the membrane potential or amplitude of action potentials among the control neurons (without expressing any exogenous gene) and four groups of neurons expressing IFP1.4, IFP2.0, iRFP and IFP2.0 with HO1 ( Supplementary Fig. 7 ). Therefore, we found no evidence that HO1 expression introduces morphological or functional changes to the primary neurons. Expressing IFP2.0 in neurons of Drosophila On the basis of these results, we then evaluated whether IFP2.0 could be used to label neuronal processes in Drosophila . Previously, it has been shown that by targeting GFP to the plasma membrane using the transmembrane domain of the human CD4 protein (CD4-GFP), significantly larger number of dendrites can be labelled than that by GFP alone [13] . We therefore created three transgenic lines: CD4-IFP2.0+HO1 (with the ‘self-cleaving’ 2A peptide sequence [14] between IFP2.0 and HO1); CD4-IFP2.0; and CD4-iRFP. All the constructs were inserted into the same genomic locus and were driven by the same driver that labels dendritic arborization (da) neurons [15] . CD4-IFP2.0+HO1 robustly labelled da neurons, including the cell body, axon and dendrites ( Fig. 2a ), with strong signal to background ratio (~10) ( Fig. 2b ). Furthermore, smaller processes like dendritic spikes (terminal protrusions found in da neurons) were also visible ( Fig. 2d,e ). Without HO1, however, the labelled da neurons had very dim cell body fluorescence (~10 times lower); and neuronal processes, including the dendrites, could not be clearly distinguished from the background ( Fig. 2c,f ). Expression of CD4-iRFP did not generate any detectable fluorescence in da neurons, even after we increased the brightness fivefold so that the unlabelled tracheal tube could be detected due to light scattering ( Fig. 2g ). The tracheal tube is known to reflect light, which has been exploited in studying phenotypic change of the tracheal system using reflected light imaging [16] . These results demonstrate that first the IFP2.0 fusion is correctly targeted to the cell membrane and is a functional fusion tag. Second, the endogenous BV concentration is low in da neurons and therefore engineering of BV biosynthesis is necessary to image neuronal processes in Drosophila . Importantly, this engineered HO1 expression had no effect on development of the animal since the transgenic line develops normally with no observable phenotypic change. Figure 2: IFP2.0 with engineered biosynthesis of the cofactor improves neuronal imaging in Drosophila larvae Cellular membrane of dendritic arborization (da) neurons labelled by ( a , d , e ) IFP2.0 fused to CD4 with expression of HO1 that produces the cofactor (CD4-IFP2.0+HO1); ( f ) CD4-IFP2.0; ( g ) CD4-iRFP. ( b ) Fluorescence intensity profile along the line in a ; the green and red arrows point to the dendrites in a . ( c ) Normalized fluorescence intensity of the cell body pointed by the yellow arrow in a and f . ( e ) Confocal image of the area (blue box) in d , with arrows pointing to dendritic spikes. Scale bar: ( a , d , f , g ), 100 μm; ( e ), 20 μm. Full size image Expressing IFP2.0 in other tissues of Drosophila We also expressed the IFP constructs in the Drosophila trachea and wing imaginal discs and observed similar results. For these experiments, we coexpressed CD8-GFP to label cell membranes with both GFP and IFP. The transgenic lines expressing HO1 in trachea and wing disc both developed normally. CD4-IFP2.0+HO1 labelled tracheal ( Supplementary Fig. 8 ) and wing disc ( Supplementary Fig. 9 ) cells strongly and the infrared fluorescence co-localized with GFP fluorescence. In contrast, the CD4-iRFP-labelled cells were not fluorescent ( Supplementary Figs 8 and 9 ), although iRFP (not fused to other proteins) was fluorescent in the tracheal tube and membrane-associated CD8-GFP fluorescence was robust ( Supplementary Fig. 8 ). These results demonstrate that the dimeric iRFP fails to label cell membranes in Drosophila using CD4-based approach, presumably because the dimerization by iRFP interferes with CD4 trafficking to the plasma membrane. Our results therefore suggest that, in contrast to iRFP, CD4-IFP2.0 fusion will be a valuable reagent in protein labelling [17] , [18] . Expressing IFP2.0 in mouse brain tumours In addition to providing an orthogonal colour for protein labelling [19] , [20] , another advantage of IFPs is its efficient light penetration for deep tissue imaging in whole animals [21] , [22] , [23] . Previously, IFPs including IFP1.4 and iRFP have been used to image the liver in intact mice. Encouraged by the robust expression in cultured neurons and glial cells, we investigated the use of IFP2.0 to image the tumours in the mouse brain. The principal challenges for this context are its requirement for the BV chromophore and the uncertain BV concentration in the brain, the presence of the skull and the deep setting of many parts of the brain. We used a glioma model for brain imaging. We first made two lentiviral constructs expressing IFP2.0+HO1 and iRFP, respectively. Then we established stable cell lines of LN229, which is a glioma cell line established from cells taken from a patient with right frontal parieto-occipital glioblastoma [24] . Orthotopic tumours were grown by implanting the cells into the right frontal lobe of a mouse brain (five mice per cell line). At the 4th week post implantation, we examined brains in whole animals for tumour fluorescence. Because the excitation and emission maxima of IFP2.0 and iRFP are similar (690/711 and 693/712 nm, respectively), we used the same excitation (675±15 nm) and emission (720±10 nm) filters for imaging. The brain tumour expressing IFP2.0+HO1 was strongly fluorescent in intact living mice ( Fig. 3a ), suggesting that the infrared fluorescence penetrates through skull efficiently [25] . Importantly, the fluorescence signal was well-localized, indicating low scattering of the infrared fluorescence [26] . By comparison, the iRFP-expressing tumour was approximately threefold dimmer ( Fig. 3a,b ). We also imaged brains that had been extracted from such animals and found that the images were consistent with the whole-animal fluorescence and that the IFP2.0+HO1-marked tumours were significantly brighter ( Fig. 3c ). Both IFP2.0 and iRFP tumours were in the right frontal lobe of the mouse brain. The brains were then sliced, which revealed similar tumour size. The brain slices were imaged by confocal microscopy, which revealed infrared fluorescent glioma cells ( Fig. 3d ). The cells expressing IFP2.0+HO1 in the brain slice were ~3 times brighter than the cells expressing iRFP ( Fig. 3d ). Without HO1, however, IFP2.0-expressing tumours had similar brightness compared with iRFP ( Supplementary Fig. 10 ). The engineering of the cofactor biosynthesis pathway thus significantly improves brain imaging in mice. On the basis of these imaging results from intact mice, extracted brains and brain slices, we conclude that IFP2.0+HO1 is significantly better (approximately threefold) than iRFP for imaging these brain tumours in intact mice. 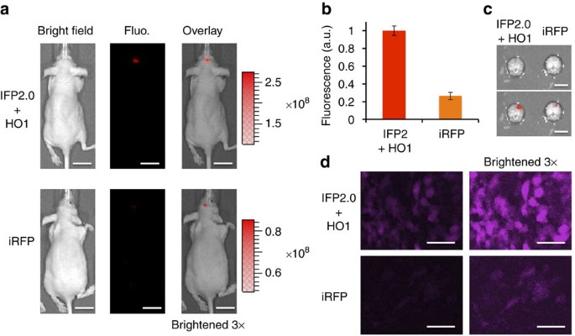Figure 3: IFP2.0 with engineered biosynthesis of the cofactor improve imaging of tumours in mice. (a) Bright field (left), fluorescence (middle) and overlay (right) images of the brain tumour (glioblastoma) in intact mice expressing IFP2.0+HO1 (top), iRFP (bottom). The fluorescence intensity in the overlay image of iRFP is threefold (3 × ) brightened compared with that of IFP2.0+HO1. The scale bar indicates fluorescence radiant efficiency. (b) Average fluorescence intensity of the brain tumour in intact mice with s.d. (c) Bright field (top) and fluorescence overlay (bottom) images of the extracted brain. (d) Confocal images of the brain slices. The right panels show 3 × brightened images. Size scale bar: (a), 1 cm; (c), 3 mm; (d), 40 μm. Figure 3: IFP2.0 with engineered biosynthesis of the cofactor improve imaging of tumours in mice. ( a ) Bright field (left), fluorescence (middle) and overlay (right) images of the brain tumour (glioblastoma) in intact mice expressing IFP2.0+HO1 (top), iRFP (bottom). The fluorescence intensity in the overlay image of iRFP is threefold (3 × ) brightened compared with that of IFP2.0+HO1. The scale bar indicates fluorescence radiant efficiency. ( b ) Average fluorescence intensity of the brain tumour in intact mice with s.d. ( c ) Bright field (top) and fluorescence overlay (bottom) images of the extracted brain. ( d ) Confocal images of the brain slices. The right panels show 3 × brightened images. Size scale bar: ( a ), 1 cm; ( c ), 3 mm; ( d ), 40 μm. Full size image We have engineered a bright monomeric IFP2.0. It is significantly brighter than IFP1.4 in cells and is similar to the dimeric iRFP. We demonstrate that IFP2.0 tagged to CD4 labels the cell membrane in da neurons and other tissues of Drosophila , whereas CD4_iRFP fusion fails to label the cell membrane. Therefore, IFP2.0 is suitable for protein labelling at infrared wavelengths, which adds an orthogonal colour to green and red FPs. IFP2.0, therefore, provides a new opportunity and dimension in the study of protein–protein and cell–cell interactions. In contrast to GFP that provides the chromophore by itself requiring only oxygen for the maturation, phytochrome-derived IFPs incorporate the endogenous molecule BV as the chromophore. We discover that in primary hippocampal neurons, the cofactor BV is limited. Engineered biosynthesis of BV significantly improved the brightness of IFP2.0, and therefore it enhances neuronal imaging using IFP2.0 as well as other IFPs. We find that BV is also limited in the da neurons in Drosophila , and that the engineered biosynthesis pathway enables us to image neuronal processes including dendrites and dendritic spikes in intact Drosophila larvae. Our method will therefore have useful applications in biological studies based on this important model organism. For example, because IFP2.0 is orthogonal to other visibly FPs, plasma membrane-targeted IFP2.0 may be used to study how neuronal circuits are established through cell–cell interactions. We also demonstrate that IFP2.0 and the engineered BV biosynthesis enable us to image brain tumour in intact mice, with significantly improved fluorescence intensity compared with iRFP. This imaging method will be useful in biomedical imaging study of glioblastoma. For example, compared with luciferase, IFP2.0 not only allows whole-body imaging but also cellular and subcellular imaging, as well as cell sorting. Therefore, IFP2.0 together with HO1 may provide an opportunity to study early events during the development of glioblastoma and to sort and identify potential precursor cells. Our method may also be used to study tumour metastasis with better spatial resolution than luciferase and visibly FPs, due to efficient penetration of infrared light through tissues. Since there are many phytochrome sequences available [27] , [28] , our structural and engineering work may serve to guide future engineering of brighter and monomeric phytochrome-derived IFPs, as well as IFPs with other photophysical and -chemical properties. Gene mutagenesis and screening Genetic libraries were constructed by DNA shuffling using IFP1.4 and IFP1.1 as substrates followed by random mutagenesis. To prepare genes to be shuffled, about 10 μg of plasmids containing IFP1.4 and IFP1.1 gene was digested at 37 °C for 1 h with BamH1 and EcoRI. Fragments of ~1 kb were purified from 1% agarose gels using zymoclean gel DAN gel recovery kit (Zymo Research). The DNA concentrations were measured and the fragments were mixed 1:1 for a total of ~2 μg. The mixture was digested with 0.5 unit DNase I (New England Biolabs) in 25 μl of 10 mM Tris-HCl (pH7.6), 2.5 mM MgCl 2 and 0.5 mM CaCl 2 at15 °C for 13 min and terminated by heating at 95 °C for 10 min. The DNase I digests were run on a 2% agarose gel, and the size of 50–100 bp fragments were cut and purified by zymoclean gel DAN gel recovery kit (Zymo Research). Ten microlitres of purified fragments was added to 10 μl Phusion High-Fidelity PCR Master Mix and reassembled with a PCR program of 30 cycles, with each cycle consisting of 95 °C for 60 s, 50 °C for 60 s and 72 °C for 30 s. After gene reassembly, 1 μl of this reaction was amplified by PCR. Shuffled mutant library was expressed in E. coli strain TOP10 and grown overnight on LB/agar (supplemented with 0.02% (wt/vol) L - arabinose (Sigma) at 37 °C and screened by imaging the agar plates with colonies using a BioSpectrum Imaging System (UVP, Upland, CA) in the APC channel (720 nm) illuminated by 690 nm light. The brightest clone of the shuffled library was used as template and subjected to four rounds of random mutagenesis. Random mutagenesis was performed with a GeneMorph II Random Mutagenesis Kit (Stratagene). Mutant libraries were expressed and screened as described above. The brightest clone in each library was picked as a template for the next round of random mutagenesis. Protein purification and characterization IFP1.4, IFP2.0 and iRFP were expressed with C-terminal polyhistidine tag on a pBAD expression vector (Invitrogen). Proteins were purified with the Ni-NTA purification system (Qiagen). Protein concentration was measured by using the BCA method (Pierce). The extinction coefficients were based on a comparison of absorbance values for the protein at the main peak (692 nm or 694 nm) with the absorbance value at the 391 nm peak assuming the latter to have the extinction coefficient of the free BV, which is 39,900 M −1 cm −1 . For determination of quantum yield, fluorescence signal of IFP2.0 was compared with that of the equally absorbing IFP1.4, iRFP and Alexa Fluor 647 dye (quantum yield is 0.33 in PBS, Invitrogen). Protein expression and purification for crystallography A 6 × His-tagged recombinant protein was expressed in E. coli CodonPlus (DE3) RIL Cells (Stratagene). One litre LB broth medium containing 1 mM Ampicillin was inoculated with 10 ml of an overnight culture at 37 °C. At an OD 600 of approximately 0.6, expression of recombinant IFP2.0 was induced by the addition of 0.02% of arabinose, and cells were grown for an additional 24 h at 37 °C. Cells were pelleted by centrifugation (4,000 g , 4 °C, 30 min), resuspended in buffer A (20 mM Tris-HCl pH 8.0, 500 mM NaCl), complemented with complete protease inhibitors-EDTA (Roche)) and disrupted using a sonicator. The soluble fraction was recovered by centrifugation (40,000 g , 4 °C, 30 min) and loaded on a 5 ml Ni-NTA superflow column (Qiagen) pre-equilibrated with buffer A. The His-tagged protein was eluted with 150 mM imidazole in buffer A. Fractions containing purified proteins were pooled and concentrated to 1 ml using Centricon devices (Amicon 30,000 Da cutoff) and loaded onto a size-exclusion chromatography column (Hiload Superdex 75, 10/300, GE Healthcare) for the final step of the purification procedure. The column was equilibrated with 20 mM Tris-HCl pH 8.0, and the pooled peak fractions were concentrated to 18 mg ml −1 . The purity of the protein solutions was confirmed by SDS-PAGE. The final concentration was determined by UV spectroscopy assuming molar absorption coefficients at 280 nm of 34,045 M −1 cm −1 . Crystallization Initial trials were performed using the sitting-drop method and commercial crystallization screening kits from Qiagen and Hampton Research. For the initial trials, we used a Cartesian PixSys 4,200 crystallization robot (Genomic Solutions, U.K.) using 96-well Greiner Crystal Quick plates (flat bottom, untreated). Protein solution of volume 0.1 μl was mixed with 0.1 μl reservoir solution and the resulting drops were equilibrated against 100 μl reservoir solution. After optimization of the conditions, the best IFP2.0 crystals grew at room temperature in 28% PEG 400, 0.1 M Sodium acetate pH 4.6. in 1–1.5 μl hanging drops using the vapour diffusion method. X-ray diffraction data collection and structure refinement Before diffraction experiments, crystals were flash-cooled directly in liquid nitrogen. X-ray diffraction experiments were performed at the European Synchrotron Radiation Facility (Grenoble, France). Data were collected at 100 K at a wavelength of 0.873 Å on beamline ID23-eh2. Diffraction data sets were processed using XDS [29] , and intensities were scaled and reduced with AIMLESS [30] . The crystal belongs to the C2 space group and diffracted to 1.14 Å resolution. The solvent content is 46%. Structure refinement was conducted with Refmac5 using anisotropic B-factors [31] . The thioether bond between Cys24 and the chromophore BV appears to be X-ray sensitive. Structure and experimental data have been deposited in the Protein Data Bank under the PDB ID 4cqh. Crystallographic data statistics can be found in Supplementary Table S2 of the Supplementary Information . Gel filtration chromatography Gel filtration chromatography was performed using a Superdex-200 HR 10/30 FPLC gel filtration column (Amersham Biosciences). The column was equilibrated with sterile PBS in a cold room. Hundred microlitres of purified proteins at a concentration of 0.5 mg ml −1 in PBS was loaded on the column. Elution was performed in PBS, at a flow rate of 0.5 ml min −1 for 45 min. The column effluent was monitored by absorbance at 280 and 630 nm. Gel filtration standard proteins of throglobulin, BSA, azurin and aprotinin were also loaded under the same conditions to calibrate the column. The linear calibration curve representing the logarithm of molecular mass as a function of the fraction number was used to calculate the molecular mass of the IFP2.0. Characterization in mammalian cells and neurons For characterization in mammalian cells, IFP1.4, IFP2.0, IFP2.0+HO1 and iRFP were cloned into pcDNA3.1 vector under CMV promoter. We also cloned GFP under internal ribosome entry site into the same vector. HEK293A cells were transfected using calcium phosphate transfection method and then imaged 48 h later on a Nikon eclipse Ti inverted epifluorescence microscope with red-shifted Cy5.5 filter set (665/45 nm exciter and 725/50 nm emitter, Chroma) and a digital CMOS camera, controlled by NIS-Element software (Nikon Instruments). Images were processed and analysed with ImageJ. The fluorescence intensity of IFPs was normalized by the fluorescence intensity of coexpressed GFP to accommodate variations in transfection efficiency among cells. For characterization in neurons, hippocampi were dissected from 19-day embryonic rats (E19), digested with a mixture of proteases at 37 °C for 15 min and dissociated with a fire-polished Pasteur pipette in plating medium (minimal essential medium (MEM) containing Earle’s salts with 10% fetal bovine serum, 0.5% glucose, 1 mM sodium pyruvate, 25 μM glutamine, and 1 × penicillin/streptomycin). Neurons were then plated onto glass coverslips (Warner Instruments) pretreated with nitric acid and coated with poly- L -lysine (0.1 mg ml −1 ; Sigma-Aldrich). Each 12-mm coverslip was plated with 5 × 10 4 neurons, which were maintained in neurobasal medium (Invitrogen) containing B27 extract (Invitrogen), 0.5 mM glutamine, 100 units of penicillin and 100 μg ml −1 of streptomycin. Neuronal culture was incubated at 37 °C with 5% CO 2. For transient transfection, neurons in culture at 9 DIV were treated with Opti-MEM containing IFP1, 4, IFP2.0, IFP2.0+HO1 or iRFP plasmid, and Lipofectamine 2,000 (Invitrogen). Images were taken 48 h after transfection. Cells were imaged on a Zeiss Axiovert microscope with a Cy5 filter set (Chroma) and a CoolSNAP ES2 CCD Camera (Photometrics, Tucson, AZ), controlled by MetaMorph software (version 7.6.2.0, Molecular Devices, Sunnyvale, CA). To perform whole-cell recording, recording pipettes were routinely filled with a solution containing 125 mM K- gluconate, 15 mM KCl, 10 mM HEPES, 3 mM MgATP, 0.3 mM Na-GTP, 5 mM Na-phosphocreatine and 0.2 mM EGTA (pH 7.2–7.4, 290–300 mosM). The cells on coverslips were placed in an oxygenated (95% O 2 and 5% CO 2 ) solution containing 119 mM NaCl, 2.5 mM KCl, 2.5 mM CaCl 2 , 1.3 mM MgSO 4 , 1 mM NaH2PO4, 26.2 mM NaHCO 3 and 11 mM glucose. Action potentials were induced by injection of currents under current clamp. Characterization in Drosophila For characterization of neuronal processes in Drosophila , CD4-IFP2.0, CD4-IFP2.0+HO1 and iRFP were cloned into pACU2 vector (Addgene). Transgenic lines of CD4-IFP2.0+HO1 (with the ‘self-cleaving’ 2A peptide sequence 15 between IFP2.0 and HO1), CD4-IFP2.0, CD4-iRFP were created by ΦC31-mediated transformation at the attP VK00019 docker site. Gal4 21-7 was used to drive the expression of the transgenes in all da neurons. For live imaging of larvae, the animals were reared at 25 °C in density-controlled vials. Third instar larvae at 96 h after egg laying were mounted in glycerol on glass slides. The dorsal da neuron cluster was imaged with a × 40 NA1.25 oil lens on a Leica SP5 confocal microscope. For excitation of IFP2.0 and iRFP, 633 nm laser was used. Images shown are maximum intensity projections of image stacks covering a da neuron layer (8–11 μm). For characterization in the Drosophila tracheal tube, Btl-Gal4:UAS-CD8GFP flies were crossed with UAS-CD4-IFP2.0 or UAS-IFP2.0 transgenic flies. The IFP2.0, IFP2.0+HO1 and iRFP plasmids are inserted into the same locus at third chromosome. For confocal imaging, flies were maintained on a cornmeal and agar medium at 25 °C according to the standard protocol. Wandering third instar larvae were collected and dissected in cold PBS. Wing imaginal discs were placed in a droplet of 1 × PBS buffer on the coverslip. The discs were gently flattened and attached to coverslips by reducing the amount of PBS. Then the coverslips were inverted on depression slides. The wing discs were hanging in the centre of depression. Images were taken on a Nikon spinning disk confocal. Construction of lentiviral vectors and cell transfection To create Lentivirus expressing IFP1.4, IFP2.0, IFP2.0+HO1 or iRFP and GFP, a transcription unit comprising the IFP1.4, IFP2.0, IFP2.0+HO1 or iRFP coding sequence, the poliovirus IRES and GFP was constructed by assembly PCR, cloned into pENTR1a (Invitrogen) and transferred into pLenti-CMV-DEST (Invitrogen) by Gateway recombinase (Invitrogen). Viruses were produced in HEK293 cells with ViraPower Lentiviral Expression System (Invitrogen) according to the manufacturer’s recommendations and purified by anion exchange chromatography (FastTrap purification kit, Millipore), resuspended in HBSS+10% glycerol and stored in aliquots at −80 °C. Titers as assessed on HEK293 cells by GFP fluorescence were 44,000 infectious units (IU) per ml for each virus. For transfection, LN229 Cells were plated on 100 mm culture dishes and cultured to ~80% confluence. Three millilitres of virus aliquots and 3 ml of fresh medium were mixed and added on the cells. Long-term transgene expression was maintained by selecting for resistance to puromycin at a final concentration of 10 μg ml −1 . Intracranial Xenografts and in vivo mouse brain imaging LN229 cells stably expressing IFP2.0, IFP2.0+HO1 or iRFP were cultured in H21 medium containing 10% FBS, harvested in logarithmic growth and suspended at a density of 2 × 10 8 cells per ml in PBS at room temperature. For intracranial injection, 4- to 6-week-old female BALB/c nu/nu mice (Harlan; Sprague–Dawley) were anaesthetized (five mice for each constructs), and a small surgical incision was made in the skin covering the skull 2 mm to the right of the bregma. Cell suspensions (5 μl) containing approximately 1 × 10 6 LN229 cells at room temperature were slowly (~6 s) injected intracranially at 3.5 mm below the skull surface using a 29-gauge needle. Immediately thereafter the incision was closed with surgical adhesive, and the animals were monitored until conscious and returned to their cages. Intracranial xenograft growth was assessed twice weekly. Tumours were established about 2 weeks after injections. All mouse experimentation was performed in accordance with protocols approved by the IACUC at the University of California, San Francisco and adhered to the National Institutes of Health Guide for the Care and Use of Laboratory Animals. Mouse imaging was performed with an IVIS Spectrum instrument (Caliper LifeSciences) in epifluorescence mode equipped with 675/30 nm and 720/20 nm filters for excitation and emission, respectively. All quantitative measurements of fluorescence signal were performed using the Living Image Software 4.0. Confocal imaging of acutely isolated brain slices Slices were prepared according to standard procedures. Mice were anaesthetized with isoflurane and decapitalized. Mouse brains were dissected rapidly and sliced (400 μM in thickness) with a vibratome (VT-1000S; Leica) in ice-cold oxygenated (95% O 2 and 5% CO 2 ) artificial cerebrospinal fluid solution (aCSF) containing 119 mM NaCl, 2.5 mM KCl, 2.5 mM CaCl 2 , 1.3 mM MgSO 4 , 1 mM NaH2PO 4 , 26.2 NaHCO 3 and 11 mM glucose. The slices were imaged on a Zeiss LSM510 confocal microscope equipped with objective × 63/0.9W (Zeiss). Slices were scanned by 633 nm laser in xyz mode with 8 μm interval between slices. Projection images were made from z-stacks. During imaging, slices were kept in a chamber with perfusion of CSF at room temperature. Accession codes : Coordinates and structure factors for IFP2.0 have been deposited in the RCSB Protein Data Bank under accession code 4cqh . How to cite this article: Yu, D. et al. An improved monomeric infrared fluorescent protein for neuronal and tumour brain imaging. Nat. Commun. 5:3626 doi: 10.1038/ncomms4626 (2014).